An energy transduction mechanism used in bacterial flagellar type III protein export Flagellar proteins of bacteria are exported by a specific export apparatus. FliI ATPase forms a complex with FliH and FliJ and escorts export substrates from the cytoplasm to the export gate complex, which is made up of six membrane proteins. The export gate complex utilizes proton motive force across the cytoplasmic membrane for protein translocation, but the mechanism remains unknown. Here we show that the export gate complex by itself is a proton–protein antiporter that uses the two components of proton motive force, Δψ and ΔpH, for different steps of the protein export process. However, in the presence of FliH, FliI and FliJ, a specific binding of FliJ with an export gate membrane protein, FlhA, is brought about by the FliH–FliI complex, which turns the export gate into a highly efficient, Δψ-driven protein export apparatus. Proton motive force (PMF), the electrochemical potential difference of protons across a biological membrane, is utilized as the energy source of many biological activities, including protein export, ATP synthesis and flagellar motor rotation. PMF consists of two components: the electric potential difference (Δψ) and the proton concentration difference (ΔpH). Although Δψ and ΔpH are equivalent driving forces for proton movement and translocation in physics and have also been believed to have equivalent roles in biological functions, recent experimental data suggest a differential usage of Δψ and ΔpH in biological processes, such as flagellar motor rotation [1] and ATP synthesis [2] . The bacterial flagellum, which is responsible for motility, consists of at least three substructures: the basal body, the hook and the filament. Flagellar assembly begins with the basal body, followed by the hook and finally the filament. For construction of the flagellum, many of the flagellar component proteins are transported to the distal end of the flagellar structure by the flagellar type III protein export apparatus. The export apparatus consists of three soluble proteins, FliH, FliI and FliJ, and six integral membrane proteins, FlhA, FlhB, FliO, FliP, FliQ and FliR [3] , [4] , [5] . These components of the export apparatus share substantial sequence and functional similarities with those of the type III secretion system of pathogenic bacteria, which directly inject virulence factors into their host cells [6] . Recently, it has become apparent that FliH, FliI and FliJ are evolutionarily related to components of F O F 1 -ATP synthase, which utilizes PMF for ATP synthesis [5] , [7] , [8] , [9] . FliI is an ATPase [10] and forms a complex with FliH and FliJ [11] , [12] , [13] . The rate of the protein export is markedly low in the absence of FliH, FliI and FliJ, although these components are not essential because flagellar formation occasionally occurs in their absence [13] , [14] , [15] , [16] . The FliH–FliI–FliJ complex binds to export substrates and chaperon–substrate complexes in the cytoplasm [17] , [18] and delivers them to the docking platform of the export gate made up of the cytoplasmic domains of FlhA and FlhB (FlhA C and FlhB C , respectively) [19] , [20] . An association of the substrate-bound FliH X –FliI 6 –FliJ ring complex with the FlhA C –FlhB C docking platform induces the initial entry of the substrate into the gate [15] , [21] . The chemical energy derived from ATP hydrolysis by FliI appears to be required for the dissociation of the FliH X –FliI 6 –FliJ ring complex from the gate [22] . The export gate complex utilizes PMF as an energy source for the unfolding and translocation of export substrates into the central channel of the flagellum [15] , [16] . Interestingly, it has been shown, albeit qualitatively, that Δψ alone is sufficient to support export in wild-type cells [16] . Thus, it remains unclear how PMF is used as the energy source. To clarify the roles of the two components of PMF in flagellar protein export, we collapsed Δψ and ΔpH separately and analysed flagellar protein export in a wild-type strain of Salmonella enterica and its Δ fliH–fliI bypass mutant whose second-site P28T mutation in FlhB recovers the export efficiency of some substrates to wild-type levels; therefore, flagellar formation increases markedly in the absence of FliH and FliI [15] . We show that the export gate uses the two components of PMF differently for protein export depending on the presence and absence of FliH and FliI. Protein–protein interactions monitored by a pull-down assay using GST affinity chromatography combined with bacterial genetics show that what is required for efficient Δψ-driven protein export of the wild-type export apparatus is not FliH and FliI themselves, but instead a specific interaction of FlhA with FliJ that is brought about by the docking of the FliH–FliI 6 ring complex to the gate. Effects of Δψ and ΔpH on flagellar protein export To investigate the role of each component of PMF on flagellar protein export in wild-type cells and a Δ fliH-fliI bypass mutant [Δ fliH-fliI flhB (P28T)], Δψ and ΔpH were collapsed individually by treatment with valinomycin in the presence of KCl [16] and by adding potassium benzoate [23] , respectively. The Δψ and ΔpH were measured using tetramethylrhodamine methyl ester (TMRM) [1] and a ratiometric pH indicator protein, pHluorin [24] , respectively. Because the hook-capping protein FlgD is one of the export substrates that are secreted at wild-type levels by the Δ fliH-fliI bypass mutant [15] , we analysed the secretion level of FlgD as a representative measure of the export activity ( Fig. 1 ). The Δψ and ΔpH measured at different pH values in the presence and absence of benzoate are shown in Figure 2 . 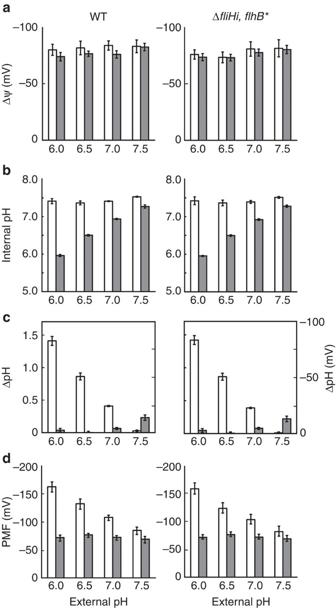Figure 2: pH dependence of PMF components. pH dependence of (a) Δψ, (b) intracellular pH, (c) ΔpH and (d) total PMF. Δψwas measured in 10 mM potassium phosphate, 0.1 mM EDTA, and 10 mM sodium lactate at an external pH of 6.0, 6.5, 7.0 or 7.5 with (closed bar) or without (open bar) 20 mM potassium benzoate using TMRM. More than 100 cells were measured. Intracellular pH was measured with pHluorin. At least six independent experiments were conducted. Vertical bars indicate standard deviations. In wild-type cells, at an external pH of 7.0, the secretion level was significantly reduced by discharging Δψ by 20 μM valinomycin at 150 mM KCl ( Fig. 1a left panel) but was not reduced at all by collapsing ΔpH by using potassium benzoate ( Fig. 1b left panel). These results confirmed a previous report [16] in a more quantitative manner. In contrast, the secretion by the Δ fliH-fliI bypass mutant was effectively abolished not only by discharging Δψ ( Fig. 1a right panel) but also by collapsing ΔpH ( Fig. 1b right panel). Interestingly, neither of the remaining ΔpH (0.35, which is equivalent to 24 mV) nor Δψ (81 mV) was effective in driving protein export. The intracellular levels of FlgD were not changed by either treatment. Because the total PMF of the fliH-fliI bypass mutant was the same as that of wild-type cells ( Fig. 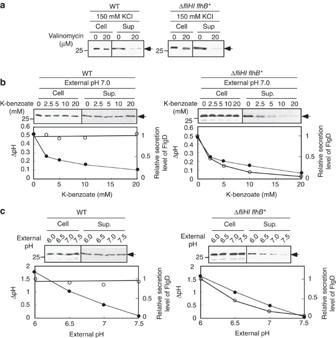2d ), these results indicate that Δψ and ΔpH are both essential and are used differently for flagellar protein export in the absence of FliH and FliI. Figure 1: Effect of Δψand ΔpH on flagellar protein export. (a) Effect of valinomycin in the presence of 150 mM KCl. Immunoblotting, using polyclonal anti-FlgD antibody, of whole-cell proteins and culture supernatant fractions prepared from SJW1103 (wild-type, indicated as WT) and MMHI0117 (ΔfliH-fliI flhB(P28T), indicated as ΔfliHI flhB*) grown at 30 °C in a buffer containing 150 mM KCl with or without 20 μM valinomycin at an external pH of 7.0. (b) Effect of potassium benzoate on the secretion level of FlgD (upper panel) and ΔpH change (closed circle) and the quantified secretion level of FlgD (open circle; lower panel) at an external pH of 7.0. Intracellular pH was measured with pHluorin. These data are the average of at least three independent measurements. The experimental errors are less than 10%. (c) Effect of external pH on FlgD secretion over a pH range of 6.0–7.5. Figure 1: Effect of Δ ψ and ΔpH on flagellar protein export. ( a ) Effect of valinomycin in the presence of 150 mM KCl. Immunoblotting, using polyclonal anti-FlgD antibody, of whole-cell proteins and culture supernatant fractions prepared from SJW1103 (wild-type, indicated as WT) and MMHI0117 (Δ fliH-fliI flhB (P28T), indicated as Δ fliHI flhB *) grown at 30 °C in a buffer containing 150 mM KCl with or without 20 μM valinomycin at an external pH of 7.0. ( b ) Effect of potassium benzoate on the secretion level of FlgD (upper panel) and ΔpH change (closed circle) and the quantified secretion level of FlgD (open circle; lower panel) at an external pH of 7.0. Intracellular pH was measured with pHluorin. These data are the average of at least three independent measurements. The experimental errors are less than 10%. ( c ) Effect of external pH on FlgD secretion over a pH range of 6.0–7.5. Full size image Figure 2: pH dependence of PMF components. pH dependence of ( a ) Δ ψ , ( b ) intracellular pH, ( c ) ΔpH and ( d ) total PMF. Δ ψ was measured in 10 mM potassium phosphate, 0.1 mM EDTA, and 10 mM sodium lactate at an external pH of 6.0, 6.5, 7.0 or 7.5 with (closed bar) or without (open bar) 20 mM potassium benzoate using TMRM. More than 100 cells were measured. Intracellular pH was measured with pHluorin. At least six independent experiments were conducted. Vertical bars indicate standard deviations. Full size image The acidification of the cytoplasm is known to interfere with flagellar protein export [16] . This relationship raised the possibility that the export apparatus of the bypass mutant may be more sensitive to low intracellular pH than the apparatus of the wild-type cells. To examine the ΔpH dependence of protein export without lowering the intracellular pH, we varied only the external pH over a range of 6.0–7.5 ( Fig. 1c ). The intracellular pH did not change significantly over this external pH range ( Fig. 2b ). In wild-type cells, the secretion level was constant over this external pH range ( Fig. 1c left panel). However, the secretion level by the Δ fliH-fliI bypass mutant showed a marked dependence on the external pH and therefore on ΔpH; it increased on a downward pH shift from 7.0 to 6.0 and almost diminished by an upward shift to 7.5 where ΔpH is nearly zero ( Fig. 1c right panel and Fig. 2c ). The Δ ψ did not change significantly over an external pH range of 6.0–7.5 ( Fig. 2a ). Because the ΔpH component of the PMF was significantly increased by lowering the external pH ( Fig. 2c ), resulting in an increase in total PMF ( Fig. 2d ), we conclude that an increase in the ΔpH component facilitates flagellar protein export in the Δ fliH-fliI bypass mutant but not in wild-type cells. We obtained essentially the same results with another fliH-fliI bypass mutant (Δ fliH-fliI flhA (V404 M)) ( Supplementary Fig. S1 ). Solvent-isotope effect on flagellar protein export We next tested whether the rate of proton transfer would affect the rate of protein export. It has been shown that D 2 O affects the high-speed rotation of the proton-driven bacterial flagellar motor at a low load because of a limitation in the rate of proton translocation through the proton channel of the stator [25] . We therefore analysed this solvent-isotope effect on the flagellar protein export. The PMF did not show any changes from replacing H 2 O with D 2 O (data not shown). Although the FlgD-secretion level of the wild-type cells was not affected by D 2 O, the secretion level of the Δ fliH-fliI bypass mutant was markedly reduced ( Fig. 3 ). Interestingly, an increase in ΔpD by lowering the external pD enhanced the secretion rate of FlgD in the bypass mutant in a manner similar to that of the ΔpH ( Fig. 3 ). This result suggests that the protein export activity is limited by the rate of proton translocation through the export gate in the absence of FliH and FliI. 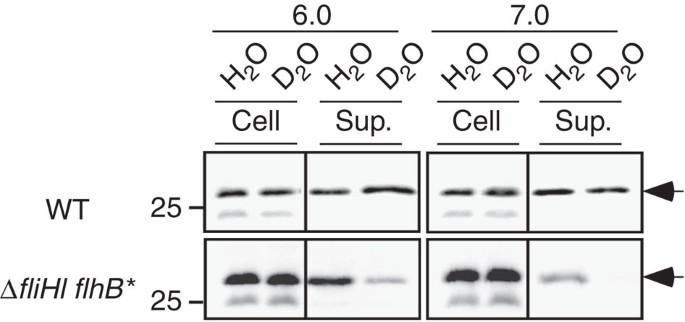Figure 3: Solvent-isotope effects on flagellar protein export. Levels of FlgD secreted by the wild-type (WT) and ΔfliH-fliI flhB(P28T) mutant (ΔfliHI flhB*) cells grown in a buffer containing either H2O or D2O at external pH levels of 6.0 and 7.0. The level of FlgD secretion was analysed by immunoblotting with the polyclonal anti-FlgD antibody. Figure 3: Solvent-isotope effects on flagellar protein export. Levels of FlgD secreted by the wild-type (WT) and Δ fliH-fliI flhB (P28T) mutant (Δ fliHI flhB *) cells grown in a buffer containing either H 2 O or D 2 O at external pH levels of 6.0 and 7.0. The level of FlgD secretion was analysed by immunoblotting with the polyclonal anti-FlgD antibody. Full size image Effect of the FlhB(P28T) mutation alone on ΔpH dependence It is thought that the flhB (P28T) mutation in the absence of FliH and FliI increases only the probability of the substrate insertion into the gate [15] . To examine the effect of this mutation by itself, we analysed the ΔpH dependence of the protein export by the flhB (P28T) mutant in the presence of FliH and FliI at an external pH of 7.0. The result was essentially the same as that of the wild-type cells; there was no ΔpH dependence ( Supplementary Fig. S2 ). This result confirms that only Δψ is used for protein export in the presence of FliH and FliI and that, when FliH and FliI are missing, the export gate requires both Δψ and ΔpH to couple the energy of the proton influx with protein export. Effect of FliJ deletion on PMF-driven protein export FliJ is required for an efficient export process, although it is not essential for export, because occasional flagellar formation is observed in its absence [14] . FliJ enhances the interaction of the FliT–FliD chaperone–substrate complex with the N-terminal portion of FlhA C [26] . Because FlhA is a component of the export gate [3] , [4] , [5] , there is a possibility that FliJ may have a role in the energy transduction mechanism of the flagellar protein export. We therefore analysed the effect of FliJ deletion in the Δ fliH-fliI bypass mutant at different external pH values. When FliJ was deleted from the Δ fliH-fliI bypass mutant, the secretion level of FlgD was largely reduced, although not to the level of the Δ fliH-fliI-fliJ triple null mutant ( Fig. 4a ). This observation indicates that the FlhB(P28T) mutation can bypass the FliJ defect to some extent. The deletion of FliJ did not change the response of the fliH-fliI bypass mutant to the change in ΔpH; a downward shift of external pH from 7.0 to 6.0 caused an increase in the secretion level both in the presence and in the absence of FliJ ( Fig. 4b ). Interestingly, co-overproduction of FliH and FliI in the Δ fliH-fliI-fliJ flhB (P28T) mutant neither bypassed the motility defect ( Fig. 4c ) nor recovered the protein export activity ( Fig. 4d ). The ΔpH dependence of the protein export remained even in the presence of FliH and FliI ( Fig. 4d ). These results clearly indicate that FliJ is the essential component responsible for the Δψ-driven protein export by the wild-type export apparatus. 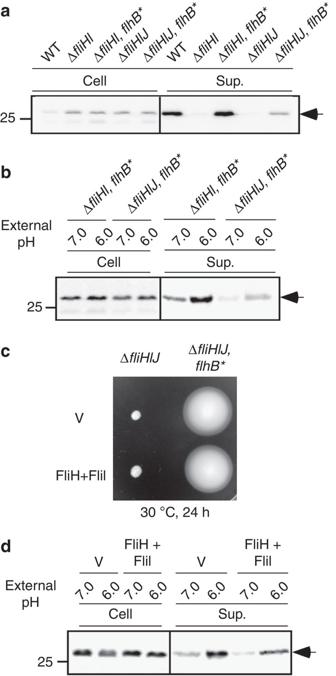Figure 4: Effects of FliJ deletion on flagellar protein export. (a) Immunoblotting, using polyclonal anti-FlgD, of whole-cell proteins and culture supernatant fractions prepared from the wild type (WT), a ΔfliH-fliIdouble null mutant (ΔfliHI), afliH-fliIbypass mutant (ΔfliHI flhB*), afliH-fliI-fliJtriple null mutant (ΔfliHIJ) and afliH-fliI-fliJ flhB(P28T) (ΔfliHIJ flhB*). (b) Effect of external pH on FlgD secretion by the ΔfliHI flhB*and ΔfliHIJ flhB*mutant strains. (c) Motility assays of MMHIJ001 (ΔfliHIJ) and MMHIJ0117 (ΔfliHIJ flhB*) transformed with pTrc99AFF4 (V) or pMMHI001 (FliH+FliI) in soft agar. The plates were incubated at 30 °C for 24 h. (d) Effect of external pH on FlgD secretion by the ΔfliH-fliI-fliJ flhB(P28T) mutant strain in the presence and absence of FliH and FliI. Immunoblotting, using polyclonal anti-FlgD antibody, of culture supernatant fractions prepared from MMHIJ0117 carrying pTrc99A or pMMHI001 grown at an external pH of 6.0 and 7.0. Figure 4: Effects of FliJ deletion on flagellar protein export. ( a ) Immunoblotting, using polyclonal anti-FlgD, of whole-cell proteins and culture supernatant fractions prepared from the wild type (WT), a Δ fliH-fliI double null mutant (Δ fliHI ), a fliH-fliI bypass mutant (Δ fliHI flhB *), a fliH-fliI-fliJ triple null mutant (Δ fliHIJ ) and a fliH-fliI-fliJ flhB (P28T) (Δ fliHIJ flhB *). ( b ) Effect of external pH on FlgD secretion by the Δ fliHI flhB *and Δ fliHIJ flhB *mutant strains. ( c ) Motility assays of MMHIJ001 (Δ fliHIJ ) and MMHIJ0117 (Δ fliHIJ flhB* ) transformed with pTrc99AFF4 (V) or pMMHI001 (FliH+FliI) in soft agar. The plates were incubated at 30 °C for 24 h. ( d ) Effect of external pH on FlgD secretion by the Δ fliH-fliI-fliJ flhB (P28T) mutant strain in the presence and absence of FliH and FliI. Immunoblotting, using polyclonal anti-FlgD antibody, of culture supernatant fractions prepared from MMHIJ0117 carrying pTrc99A or pMMHI001 grown at an external pH of 6.0 and 7.0. Full size image Interaction of FlhA with the soluble proteins FlhA is composed of an amino-terminal transmembrane domain (FlhA TM ) and a carboxy-terminal cytoplasmic domain (FlhA C ). FlhA C not only forms part of the docking platform for the soluble export components FliI, FliH and FliJ but also is directly involved in the early process of protein export with these soluble components [11] , [21] . An in-frame deletion of residues 328–351 of FlhA, which is part of the flexible linker between FlhA TM and FlhA C [27] , results in a loss-of-function phenotype [28] . It has been shown that FliJ binds to the flexible linker [26] , raising the possibility that the loss-of-function phenotype of the FlhA(Δ328–351) mutant could result from its impaired ability to interact with FliJ. However, it is not yet known whether the linker of FlhA is also involved in the interaction with FliH and FliI. To test for this possibility, we performed pull-down assays by GST affinity chromatography. We used GST as a negative control. His-FLAG-FlhA copurified with GST-FliH, GST-FliI and GST-FliJ, but not with GST alone ( Fig. 5a left panels). His-FLAG-FlhA bound to FliJ with an affinity much higher than its affinity to FliH and FliI. The deletion of residues 328–351 abolished the interaction with FliJ but not with FliH or FliI ( Fig. 5a right panels). These results indicate that residues 328–351 of FlhA are the binding target of FliJ but are not the binding target of FliH and FliI. 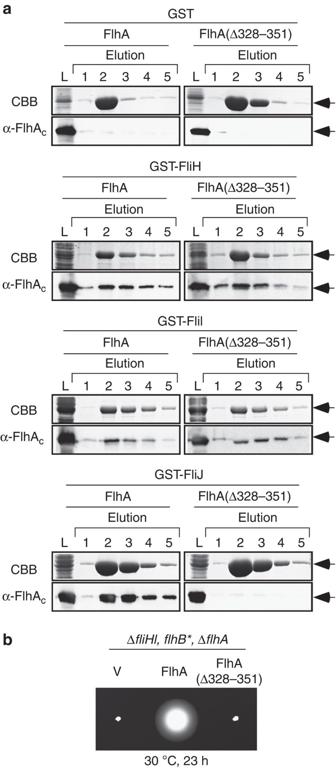Figure 5: Effect of a deletion of residues 328–351 of FlhA on the interaction with the soluble proteins. (a) Pull-down assays by GST affinity chromatography. The mixture of the soluble fractions (L) prepared from a ΔflhDC-cheWmutant expressing GST (first row), GST-FliH (second row), GST-FliI (third row) or GST-FliJ (forth row) with those from a ΔflhAmutant transformed with pMM108 (N-His-FLAG-FlhA, FlhA) or pMM108-1 (N-His-FLAG-FlhA(Δ328–351), FlhA(Δ328–351)) were loaded onto a GST column. After extensive washing, the proteins were eluted with a buffer containing 10 mM reduced glutathione. The eluted fractions were analysed by CBB staining for GST fusion proteins (upper panels) and immunoblotting with polyclonal anti-FlhA antibody (lower panels). (b) Effect of a ΔfliH-fliIbypass mutation, FlhB(P28T), on the FlhA(Δ328–351) mutants. Motility of NH0004 (ΔflhAΔfliH-fliI flhB(P28T)) transformed with pTrc99A (V), pMM108 (FlhA) or pMM108-1 (FlhA(Δ328–351)) in soft agar plate. Plates were incubated at 30 °C for 23 h. Figure 5: Effect of a deletion of residues 328–351 of FlhA on the interaction with the soluble proteins. ( a ) Pull-down assays by GST affinity chromatography. The mixture of the soluble fractions (L) prepared from a Δ flhDC-cheW mutant expressing GST (first row), GST-FliH (second row), GST-FliI (third row) or GST-FliJ (forth row) with those from a Δ flhA mutant transformed with pMM108 (N-His-FLAG-FlhA, FlhA) or pMM108-1 (N-His-FLAG-FlhA(Δ328–351), FlhA(Δ328–351)) were loaded onto a GST column. After extensive washing, the proteins were eluted with a buffer containing 10 mM reduced glutathione. The eluted fractions were analysed by CBB staining for GST fusion proteins (upper panels) and immunoblotting with polyclonal anti-FlhA antibody (lower panels). ( b ) Effect of a Δ fliH-fliI bypass mutation, FlhB(P28T), on the FlhA(Δ328–351) mutants. Motility of NH0004 (Δ flhA Δ fliH-fliI flhB (P28T)) transformed with pTrc99A (V), pMM108 (FlhA) or pMM108-1 (FlhA(Δ328–351)) in soft agar plate. Plates were incubated at 30 °C for 23 h. Full size image The P28T mutation of FlhB overcomes the FliH–FliI–FliJ defects to some extent ( Fig. 4a ). To investigate whether the P28T mutation also suppresses the FlhA(Δ328–351) defect, we transformed a Δ fliH-fliI flhB (P28T) Δ flhA mutant strain with pTrc99A, pMM108 (His-FLAG-FlhA) or pMM108-1 (His-FLAG-FlhA(Δ328–351)) and analysed the motility of the resulting transformants in soft agar plates ( Fig. 5b ). His-FLAG-FlhA restored the motility of the Δ fliH-fliI flhB (P28T) Δ flhA mutant, whereas His-FLAG-FlhA(Δ328–351) did not. This result indicates that residues 328–351 of FlhA are critical for the FlhA function even in the Δ fliH-fliI bypass mutant. Together with the binding of FliJ to residues 328–351 of FlhA ( Fig. 5a ), these results suggest that a specific conformation of the FlhA linker must be brought about by the proper binding of FliJ to residues 328–351 of FlhA to turn the export gate into an efficient, Δψ-driven protein export apparatus. Characterization of a fliJ (Δ13–24) mutant It has been shown that in-frame deletion of residues 13–24 in FliJ considerably reduced the export activity [14] . This raised the possibility that the deletion may affect the interaction with the linker region of FlhA. To test this possibility, we analysed the interaction between FlhA and FliJ(Δ13–24) by pull-down assays. His-FLAG-FlhA did not copurify with GST-FliJ(Δ13–24) ( Fig. 6a ). Unlike wild-type FliJ, FliJ(Δ13–24) did not restore motility of the Δ fliH-fliI-fliJ flhB (P28T) mutant ( Fig. 6b ). These results indicate that the reduced export activity of the fliJ (Δ13–24) mutant results from the impaired ability of FliJ to interact with the linker of FlhA. 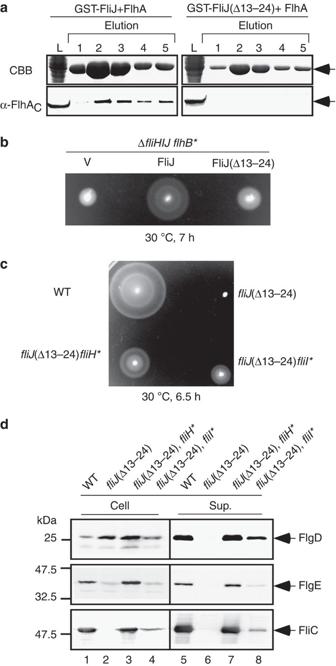Figure 6: Effects of a deletion of residues 13–24 in FliJ on the FliJ–FlhA interaction. (a) Pull-down assays by GST affinity chromatography. The eluted factions of GST-FliJ or GST-FliJ(Δ13–24) were analysed by CBB staining (upper panels), whereas the eluted FlhA protein was detected by immunoblotting with polyclonal anti-FlhA antibody. (b) Motility of a ΔfliH-fliI-fliJ flhB(P28T) (ΔfliHIJ flhB*) mutant transformed with pTrc99AFF4 (V), pMM404 (FliJ) or pRCJ104 (FliJ(Δ13–24)) in soft agar. The plates were incubated at 30 °C for 7 h. (c) Motility of pseudorevertants from thefliJ(Δ13–24) mutant: wild type (WT),fliJ(Δ13–24) mutant and its pseudorevertants (fliJ(Δ13–24),fliH(Δ96–97) (labelled asfliH*) andfliJ(Δ13–24),fliI(L244R) (labelled asfliI*)). (d) Secretion analysis of FlgD, FlgE and FliC. Immunoblotting, using polyclonal anti-FlgD, anti-FlgE or anti-FliC antibody of whole cell (Cell) and culture supernatant (Sup) fractions prepared from the above strains. Figure 6: Effects of a deletion of residues 13–24 in FliJ on the FliJ–FlhA interaction. ( a ) Pull-down assays by GST affinity chromatography. The eluted factions of GST-FliJ or GST-FliJ(Δ13–24) were analysed by CBB staining (upper panels), whereas the eluted FlhA protein was detected by immunoblotting with polyclonal anti-FlhA antibody. ( b ) Motility of a Δ fliH-fliI-fliJ flhB (P28T) (Δ fliHIJ flhB *) mutant transformed with pTrc99AFF4 (V), pMM404 (FliJ) or pRCJ104 (FliJ(Δ13–24)) in soft agar. The plates were incubated at 30 °C for 7 h. ( c ) Motility of pseudorevertants from the fliJ (Δ13–24) mutant: wild type (WT), fliJ (Δ13–24) mutant and its pseudorevertants ( fliJ (Δ13–24), fliH (Δ96–97) (labelled as fliH *) and fliJ (Δ13–24), fliI (L244R) (labelled as fliI *)). ( d ) Secretion analysis of FlgD, FlgE and FliC. Immunoblotting, using polyclonal anti-FlgD, anti-FlgE or anti-FliC antibody of whole cell (Cell) and culture supernatant (Sup) fractions prepared from the above strains. Full size image To understand the role of the specific interaction between FliJ and the flexible linker of FlhA in more detail, nine gain-of-function mutants were isolated from the fliJ (Δ13–24) mutant. Genetic mapping and DNA sequencing revealed that the second-site mutations are located in the fliH and fliI genes ( Supplementary Fig. S3 ). These pseudorevertants significantly improved motility although not as well as that of the wild type ( Fig. 6c ). Most of the flagellar proteins were detected in the culture supernatant of the pseudorevertants ( Fig. 6d ). In one of the pseudorevertants, MM104H-3 ( fliJ (Δ13–24) fliH (Δ96–97)), flagellar proteins were secreted at effectively wild-type levels ( Fig. 6d lanes 5 and 7). Consistently, the flagellar hook basal bodies, often with filaments attached, were observed by electron microscopy (data not shown). To test whether these second-site FliH and FliI mutations also suppress the fliJ -null mutant, we analysed the motility of the Δ fliH-fliI-fliJ triple null mutant transformed with pMMHI001 (FliH+FliI), pMMHI104-3 (FliH(Δ96–97)+FliI) or pMMHI104-6 (FliH+FliI(L244R)). These plasmids did not restore the motility of the Δ fliH-fliI-fliJ triple null mutant at all ( Supplementary Fig. S4a ), indicating that the second-site mutations do not suppress the fliJ -null mutation. To test the effect of each second-site mutation by itself on the motility, we isolated the second-site fliH and fliI mutants and analysed their motility. The motility was normal ( Supplementary Fig. S4b ). As these second-site mutations show no phenotype, they do not appear to affect the function of the FliH and FliI proteins. Interaction of FliJ(Δ13–24) with FliH and FliI The fliJ (Δ13–24) mutant caused six extragenic suppressors in FliH and three extragenic suppressors in FliI, raising the possibility that the deletion also affects the interaction with FliH and FliI. Therefore, we analysed the interaction of FliJ(Δ13–24) with FliH and FliI by pull-down assays. FliJ(Δ13–24) retained the ability to interact with FliH at wild-type levels and with FliI to an appreciable degree, although not at wild-type levels ( Fig. 7a ). This observation indicates that the deletion also weakens the FliJ–FliI interaction but not the FliJ–FliH interaction. The suppressor mutations in FliH and FliI did not significantly increase their binding affinity for FliJ(Δ13–24) ( Fig. 7b ). To test whether the same mutations influence the interaction of FliJ(Δ13–24) with FlhA, we analysed the interaction between FliJ(Δ13–24) and FlhA in the presence of the suppressor variants of the FliH–FliI complex. The suppressor mutation significantly improved the interaction of FliJ(Δ13–24) with FlhA ( Fig. 7c ). 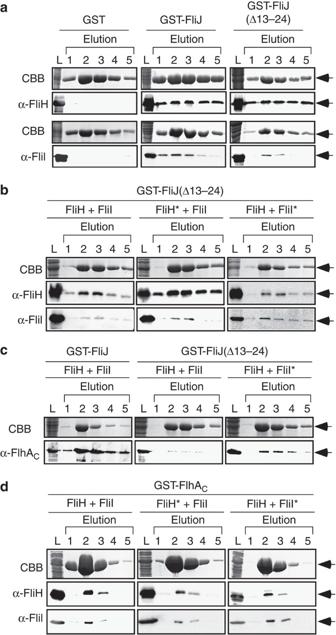Figure 7: Effect of the FliH and FliI suppressor mutations on the interaction of FliJ(Δ13–24) with FlhA. (a) Interactions of FliJ with FliH and FliI. Pull-down assays by GST affinity chromatography. The mixture of the soluble fractions (L) prepared from a ΔflhDC-cheWmutant expressing GST (left), GST-FliJ (middle) or GST-FliJ(Δ13–24) (right) with those from the ΔflhDC-cheWmutant producing His-FliH or His-FliI were loaded onto a GST column. After extensive washing, proteins were eluted with a buffer containing 10 mM reduced glutathione. (b) Interaction of GST-FliJ(Δ13–24) with the wild-type FliH–FliI complex (left) and its suppressor mutant variants (middle, FliH(Δ96–97)+FliI; right, FliH+FliI(L244R)). (c) Interactions of GST-FliJ(Δ13–24) with FlhA in the presence of a suppressor mutant variant of the FliH–FliI complex (FliH+FliI(L244R)). (d) Interaction of GST-FlhACwith the suppressor mutant variants of FliH and FliI (FliH*, FliH(Δ96–97); FliI*, FliI(L244R)). The eluted fractions were analysed by CBB staining for GST fusion proteins (upper panels) and immunoblotting with polyclonal anti-FliH, anti-FliI or anti-FlhACantibody (lower panels). Figure 7: Effect of the FliH and FliI suppressor mutations on the interaction of FliJ(Δ13–24) with FlhA. ( a ) Interactions of FliJ with FliH and FliI. Pull-down assays by GST affinity chromatography. The mixture of the soluble fractions (L) prepared from a Δ flhDC-cheW mutant expressing GST (left), GST-FliJ (middle) or GST-FliJ(Δ13–24) (right) with those from the Δ flhDC-cheW mutant producing His-FliH or His-FliI were loaded onto a GST column. After extensive washing, proteins were eluted with a buffer containing 10 mM reduced glutathione. ( b ) Interaction of GST-FliJ(Δ13–24) with the wild-type FliH–FliI complex (left) and its suppressor mutant variants (middle, FliH(Δ96–97)+FliI; right, FliH+FliI(L244R)). ( c ) Interactions of GST-FliJ(Δ13–24) with FlhA in the presence of a suppressor mutant variant of the FliH–FliI complex (FliH+FliI(L244R)). ( d ) Interaction of GST-FlhA C with the suppressor mutant variants of FliH and FliI (FliH*, FliH(Δ96–97); FliI*, FliI(L244R)). The eluted fractions were analysed by CBB staining for GST fusion proteins (upper panels) and immunoblotting with polyclonal anti-FliH, anti-FliI or anti-FlhA C antibody (lower panels). Full size image Because FliH and FliI directly bind to FlhA C [21] , it is also possible that extragenic suppressor mutations in FliH or FliI might strengthen the FliH–FlhA or FliI–FlhA interaction, respectively, so that the FliJ–FlhA interaction becomes less critical. To test this possibility, we performed pull-down assays. FliH(Δ96–97) and FliI(L244R) both copurified with GST- FlhA C at the wild-type levels ( Fig. 7d ), ruling out this possibility. Therefore, we suggest that the pseudorevertants with the second-site mutations are compensating for the FliJ(Δ13–24) mutation by altering the binding interface between FliJ and the linker of FlhA. The translocation of proteins across biological membranes requires protein transport machineries that convert biological energies into the mechanical work required for unidirectional protein transport. Nearly all the protein transport systems utilize free energy derived from cycles of nucleoside triphosphate binding and hydrolysis. In addition, PMF contributes to the driving force for protein transport across the bacterial cytoplasmic membrane, the mitochondrial inner membrane and so on [29] . However, the mechanisms of protein translocation across biological membranes by PMF remain obscure. It is thought that Δ ψ drives the translocation of negatively charged residues of preproteins across the membrane by an electrophoretic mechanism [30] , [31] , [32] . In contrast, PMF functions on the membrane components of the protein translocation machinery, altering an interaction with SecA ATPase, which uses the energy of ATP binding and hydrolysis to drive preprotein translocation into and across the cytoplasmic membrane [33] , [34] , [35] . Recently, it has been shown that the SecD/SecF complex utilizes PMF to function in the later ATP-independent stages of protein translocation [36] . In mitochondria, where Δ ψ is the dominant driving force because of its high-level generation during aerobic respiration, the inside negative potential can exert an electrophoretic effect on positively charged polypeptides that are inserted into the membrane. Δ ψ also activates an inner membrane protein channel of the mitochondrial presequence translocase [37] . Interestingly, it has been shown that Δ ψ can catalyse protein unfolding during protein translocation [38] . Thus, PMF appears to have multiple roles in protein translocation across the biological membranes. In this study, we have shown that Δ ψ alone is sufficient for flagellar protein export in wild-type cells, but both Δ ψ and ΔpH become essential in the absence of FliH and FliI ( Fig. 1 ). These results indicate that the two components of PMF have distinct roles in the flagellar protein export process in the absence of FliH and FliI. This indication suggests that a step of the Δ ψ -dependent export process is different from that powered by ΔpH. The replacement of H 2 O by D 2 O reduced the level of FlgD secretion in the absence of FliH and FliI but did not reduce it in the wild-type cells ( Fig. 3 ). Lowering the external pD value from 7.0 to 6.0 increased the secretion levels of FlgD in the absence of FliH and FliI ( Fig. 3 ), indicating that the rate of proton transfer through the export gate determines the overall rate of flagellar protein export by the export gate alone. Taken together, we propose that the flagellar type III export gate complex made up of the six membrane proteins is intrinsically a proton–protein antiporter that requires both Δ ψ and ΔpH as the energy source. Proton transport could be an intrinsic aspect of the mechanism, which is not rate determining in the wild-type export apparatus. This possibility suggests a specific structural mechanism for the essential requirement of both components of the PMF to drive protein export, although the necessary structural information is currently not available. The deletion of FliJ in addition to the deletion of FliH and FliI further reduced the level of export activity by the export gate but did not alter the ΔpH-dependent characteristics of the fliH-fliI bypass mutant ( Fig. 4b ). The export gate still requires ΔpH even in the presence of FliH and FliI when FliJ is missing ( Fig. 4d ). An increase in the ΔpH component of PMF significantly facilitated flagellar protein export in the Δ fliH-fliI-fliJ flhB (P28T) mutant ( Fig. 4b ). Therefore, FliJ appears to be required for the full activation of the export gate complex for efficient, Δ ψ -driven protein export. The FliJ–FlhA interaction with residues 328–351 of FlhA in its linker region and residues 13–24 of FliJ was found to be critical for efficient protein export ( Figs. 5 and 6 ). Because the fliJ (Δ13–24) suppressor mutations in FliH or FliI significantly improved the impaired ability of FliJ(Δ13–24) to interact with the linker of FlhA ( Figs. 6 and 7 ), we propose that FliJ requires support of FliH and FliI to efficiently and properly interact with the linker of FlhA to switch the conformation of the export gate complex into the Δ ψ -driven mode, which appears to be much more efficient than the export gate made up of the six membrane proteins by themselves. The flhB (P28T) mutation restored motility of the Δ fliH-fliI-fliJ triple null mutant to some degree ( Fig. 4 ) but not that of the Δ fliH-fliI flhA (Δ328–351) mutant ( Fig. 5 ), indicating that the linker region of FlhA is essential for flagellar protein export. We propose that a specific conformation of the FlhA linker region brought about by the proper binding of FliJ is critical for the efficient, Δ ψ -driven energy transduction mechanism of flagellar protein export. It has been proposed that FliJ is not only a general chaperone to prevent premature aggregation of export substrates in the cytoplasm [14] but also a chaperone escort protein that promotes the cycling of substrate-specific chaperones, FlgN and FliT [39] . The present study, however, has made it clear that FliJ is directly involved in a critical energy-transduction process with FlhA. FliJ facilitates FliI ring formation by binding to the centre of the ring, thereby stimulating the ATPase activity [9] , [39] . ATP hydrolysis by FliI promotes the disassembly of the FliI ring, presumably for the rapid turnover of the process of substrate delivery and insertion to the export gate [15] , [22] . Because FliJ binds to the linker of FlhA to fully activate the Δ ψ -driven protein export by the export gate ( Fig. 5 ), we propose that FliJ is a key protein that switches the export gate, which by itself is a low-efficient proton–protein antiporter, into a highly efficient, Δ ψ -driven protein export apparatus. Thus, 'export gate-activator switch' would be a more appropriate name for FliJ. Why is Δ ψ alone sufficient for protein export in wild-type cells? It has been shown that the flagellar export apparatus is evolutionarily related to F o F 1 -ATPsynthase, which utilizes PMF and ATP for ATP synthesis and proton pumping, respectively [5] . Although the structural mechanism of the flagellar type III protein export apparatus remains obscure, that of F o F 1 -ATPsynthase is well characterized: the α/β subunits form the α 3 β 3 hexameric ring as the core domain of F 1 ; the γ subunit forms the central stalk connecting F 1 with F o and is rotated within the central hole of the α 3 β 3 ring by the PMF-driven rotation of the F o ring in the membrane; the b and δ subunits form the peripheral stalk connecting F 1 with F o , to function as the stator [40] . In many of these aspects, the export apparatus shows similarities with F o F 1 -ATPsynthase: FliI forms a homo-hexamer ring to exert its ATPase activity [41] , [42] ; the structures of FliI and FliJ show extensive structural similarity to the α/β subunits [8] and the γ subunit [9] , respectively; FliJ binds to the centre of the FliI ring in a manner similar to the antiparallel α-helical-coiled coil formed by the N- and C-terminal regions of the γ-subunit penetrating into the central cavity of the α 3 β 3 ring [9] ; the amino-acid sequences of the N- and C-terminal regions of FliH are homologous to those of the b and δ subunits, respectively [7] ; the export gate complex made up of the six integral membrane proteins is powered by PMF across the cytoplasmic membrane [15] , [16] . Taken together, it may be possible that the export gate complex utilizes free energy derived from ATP hydrolysis by the FliH X -FliI 6 -FliJ ring complex for efficient proton translocation through the proton channel of the gate complex. Because the export gate by itself functions as a proton–protein antiporter, the proton translocation mechanism of the gate may also be similar to that of F o F 1 -ATPsynthase. However, because the present study has clearly shown that one of the important roles of the FliH–FliI ring complex is to bring FliJ to the FlhA linker region to switch the export gate from a low-efficient proton–protein antiporter to a highly efficient, Δ ψ -driven protein export apparatus, the structural similarity between the two systems in their entire assemblies may be used solely to achieve distinct mechanisms for their distinct functions. The detailed structural information of the entire export apparatus is essential for the mechanistic understanding of the flagellar protein export process in detail. Bacterial strains and media Salmonella strains and plasmids used in this study are listed in Table 1 . L-broth (LB) and soft tryptone agar plates were prepared as described in refs 11 , 43 . Motility medium contained 10 mM potassium phosphate, 0.1 mM EDTA and 10 mM sodium lactate. The pH value of each motility medium was adjusted to the desired pH by the addition of HCl or KOH in the presence or absence of potassium benzoate. Ampicillin was added to LB to a final concentration of 100 μg ml −1 . Table 1 Strains and plasmids used in this study. Full size table DNA manipulations and transductional crosses DNA manipulations were performed as described before [28] . P22-mediated transductional crosses were performed with p22HT int as described in ref. 44 . Construction of the Salmonella deletion mutants A Δ fliH-fliI-fliJ triple null mutant and a Δ fliH-fliI-fliJ flhB (P28T) mutant were constructed using the λ-red homologous recombination system [45] . Motility assay Fresh colonies were inoculated on soft tryptone agar plates and incubated at 30 °C. At least five independent experiments were conducted. Secretion assay The cells were grown with shaking in 5 ml of LB at 30 °C until the cell density had reached an OD 600 of ~1.0 and were washed twice with the motility buffer at pH 7.0. To test the effect of Δ ψ on flagellar protein export, we used valinomycin as described in ref. 16 . To test the effects of ΔpH on the export, the cells were resuspended in the 5-ml motility buffer at pH 6.0, 6.5, 7.0 or 7.5 in the presence and absence of potassium benzoate and incubated at 30 °C for 1 h. To test the D 2 O effect, the cells were resuspended in the 5-ml motility buffer prepared in D 2 O and incubated at 30 °C for 1 h. Cultures were centrifuged to obtain cell pellets and culture supernatants. Cell pellets were resuspended in the SDS-loading buffer, followed by normalization to a cell density to yield a constant amount of cells. Proteins in the culture supernatants were precipitated using 10% trichloroacetic acid, suspended in the Tris/SDS loading buffer and heated at 95 °C for 5 min. After SDS–PAGE, immunoblotting with polyclonal anti-FlgD, anti-FlgE and anti-FliC antibodies was performed as described before [43] . Detection was performed with an ECL immunoblotting detection kit (GE Healthcare). At least three independent secretion assays were performed. Measurement of the membrane potential The membrane potential was measured as described by Lo et al . [1] . Cells were suspended in motility medium plus 10 mM EDTA for 20 min. Cells were washed with motility medium and incubated in motility medium containing 0.1 μM TMRM (Invitrogen) for 10 min at room temperature. To observe bacterial cell bodies and epifluorescence of TMRM, we used an inverted fluorescence microscope (IX-71, Olympus) with a ×150 oil immersion objective lens (UApo150XOTIRFM, NA 1.45, Olympus) and an electron-multiplying charged-coupled device camera (C9100-02, Hamamatsu Photonics), as described before [46] . Calculation of the membrane potential was performed as described in ref. 1 , with minor modifications. More than 100 wild-type cells and a fliH-fliI bypass mutant were measured at various external pH values with or without 20 mM potassium benzoate. Intracellular pH measurement Intracellular pH measurements of wild-type cells and a Δ fliH-fliI bypass mutant transformed with pYVM001, which encodes pHluorin(M153R) on pKK223-3 (ref. 47 ), were recorded at various external pH values with or without potassium benzoate, as described previously [48] . The fluorescence-excitation spectra of the wild-type and Δ fliH-fliI bypass mutant cells expressing pHluorin(M153R) were recorded on a fluorescence spectrophotometer (RF-5300PC, Shimadzu). The 410/470-nm excitation ratios were calculated and converted to pH values based on the calibration curve. At least six independent measurements were recorded. Pull-down assays by GST affinity chromatography The soluble fractions prepared from SJW1364 (Δ flhDC-cheW ) expressing GST-FliH, GST-FliI, GST-FliJ, GST-FliJ(Δ13–24) or GST-FlhA C were mixed with those from the Δ flhDC-cheW mutant transformed with pMM108 (His-FLAG-FlhA), pMM108-1 (His-FLAG-FlhA(Δ328–351)), pMM306 (His-FliH), pMM1702 (His-FliI), pMM406 (His-FliJ), pMMHI001 (FliH+FliI), pMMHI104-3 (FliH(Δ96–97)+FliI) or pMMHI104-6 (FliH+FliI(L244R)) were loaded onto a glutathione Sepharose 4B column (bed volume, 1 ml; GE Healthcare). After the column was extensively washed with 25 ml of PBS (8 g of NaCl, 0.2 g of KCl, 3.63 g of Na 2 HPO 4 ·12H 2 O, 0.24 g of KH 2 PO 4 , pH 7.4, per litre), proteins were eluted with 50 mM Tris-HCl, pH 8.0, and 10 mM reduced glutathione. Fractions containing GST, GST-FliH, GST-FliI, GST-FliJ, GST-FliJ(Δ13–24) or GST-FlhA C were identified by SDS–PAGE with Coomassie brilliant blue (CBB) staining and immunoblotting with polyclonal anti-FlhA C , anti-FliH or anti-FliI antibody. Detection was performed with an ECL immunoblotting detection kit (GE Healthcare). At least three independent pull-down assays were performed. How to cite this article: Minamino, T. et al . An energy transduction mechanism used in bacterial flagellar type III protein export. Nat. Commun. 2:475 doi: 10.1038/ncomms1488 (2011).